Structural basis for cellobiose dehydrogenase action during oxidative cellulose degradation A new paradigm for cellulose depolymerization by fungi focuses on an oxidative mechanism involving cellobiose dehydrogenases (CDH) and copper-dependent lytic polysaccharide monooxygenases (LPMO); however, mechanistic studies have been hampered by the lack of structural information regarding CDH. CDH contains a haem-binding cytochrome (CYT) connected via a flexible linker to a flavin-dependent dehydrogenase (DH). Electrons are generated from cellobiose oxidation catalysed by DH and shuttled via CYT to LPMO. Here we present structural analyses that provide a comprehensive picture of CDH conformers, which govern the electron transfer between redox centres. Using structure-based site-directed mutagenesis, rapid kinetics analysis and molecular docking, we demonstrate that flavin-to-haem interdomain electron transfer (IET) is enabled by a haem propionate group and that rapid IET requires a closed CDH state in which the propionate is tightly enfolded by DH. Following haem reduction, CYT reduces LPMO to initiate oxygen activation at the copper centre and subsequent cellulose depolymerization. The need for renewable energy is increasing rapidly, and biofuel derived from plant matter is an attractive alternative to fossil-based fuels. However, the bioconversion of the major component of plant matter, cellulose, to low-molecular-weight saccharides is problematic and costly [1] , [2] . Despite decades of research on the molecular mechanisms of microbial cellulose depolymerization, a comprehensive picture of this elaborate biodegradation machinery has remained elusive. In nature, rot fungi and bacteria are primary factors in the recycling of lignocellulose-based biomass, and the efficient saccharification of cellulose has historically been assigned to a cascade of hydrolytic enzymes. An oxidative system was recently discovered in which extracellular flavocytochromes, that is, cellobiose dehydrogenases (CDHs) [3] , [4] , [5] , [6] , [7] , cooperate with copper-dependent lytic polysaccharide monooxygenases (LPMOs) [8] , [9] , [10] , [11] , [12] , [13] to catalyse redox-mediated glycosidic bond cleavage in crystalline cellulose, hemicelluloses and starch. The CDH-LPMO system enhances the degradation efficiency of crystalline regions in cellulose by a previously unknown mechanism [14] , [15] , [16] , [17] , [18] , [19] . CDHs are large flavocytochromes containing a haem b -binding cytochrome domain (CYT) connected by a long, flexible linker to a flavin adenine dinucleotide (FAD)-binding dehydrogenase domain (DH) [20] . Class-I CDHs are produced by basidiomycetes and lack additional domains, whereas class-II CDHs occur in ascomycetes either with or without a type-1 carbohydrate-binding module (CBM), corresponding to classes IIA and IIB, respectively [20] , [21] . Despite the absence of a CBM, class-I CDHs bind strongly to the cellulose surface by an unknown mechanism [22] . The DH domain oxidizes cellobiose at the C1 position to cellobiono-1,5-lactone with reduction of FAD. The ensuing step involves inter-domain electron transfer (IET) from the reduced FAD to CYT haem b , presumably by single electron-transfer (ET) events, followed by ET from CYT to external electron acceptors [20] such as LPMOs. LPMOs directly hydroxylate the crystalline polysaccharide substrate at C1 or C4 to produce the aldonic acid or the 4-keto sugar, respectively [10] , [17] . The precise mechanism of the monooxygenation reaction is unknown but likely involves C-H activation in which hydrogen abstraction and the formation of a radical oxygen species enable substrate hydroxylation, either by a superoxo mechanism [15] , [17] , [23] or by an oxyl mechanism [24] . As the linker between CYT and DH is long and flexible, attempts to crystallize full-length CDHs have been unsuccessful. For the CDH from the basidiomycete Phanerochaete chrysosporium ( Pc CDH), crystal structures of the proteolytically generated CYT and DH fragments were determined separately [25] , [26] , but these studies did not provide experimental information regarding the physical association between CYT and DH. The lack of full-length CDH structures has also hampered analysis of the possible mechanisms for ET between CDH and external electron acceptors such as LPMOs. Here we report the crystal and solution structures of open and closed states of two fungal CDHs and one LPMO. The closed CDH structure reveals a shielded IET pathway from FAD in the DH domain to the haem b in the CYT domain. Haem propionate-A in CYT enters the DH active site to interact with four side chains that we refer to as the propionate-docking site on DH. To evaluate whether this closed structure represents the relevant conformational state for productive IET, we performed rational site-directed mutagenesis of selected residues positioned between the FAD cofactor and the haem propionate-A, as well as rapid-kinetics measurements, to probe IET between FAD and haem b in the CDH variants. By applying small-angle X-ray scattering to deglycosylated and glycosylated forms of CDH in the absence and presence of an inhibitor, we demonstrated that both the open and closed CDH states are represented in solution. We also show, for the first time, direct and rapid ET between CYT and LPMO, and that DH is unable to transfer electrons to LPMO. Our CDH crystal structures provide a necessary structural platform for further studies on the interaction mechanism between CDH and LPMO during cellulose depolymerization. Crystal structures of the closed and open states of CDH We screened a range of basidiomycete and ascomycete fungi and ultimately achieved successful crystallization and structure determination of two full-length CDHs from the ascomycetes Myriococcum thermophilum ( Mt CDH) and Neurospora crassa ( Nc CDH) ( Fig. 1 ), and of LPMO 9F from N. crassa . The crystal structure of Mt CDH was determined at 3.2 Å and revealed a closed state in which the CYT domain is docked onto the DH domain in an arrangement that would allow efficient IET from FAD to haem b ( Fig. 2a ). In the closed IET-competent state, the haem b propionate-A stretches into the active-site pocket in DH, where the propionate carboxyl group forms an anion–quadrupole interaction with the electropositive edge of the Trp295 benzene ring ( Fig. 2a ). Propionate-A engages in an ionic interaction with Arg698, which stabilizes the propionate in its ionized state. The haem b propionate-D is folded away, and a hydrogen bond to Tyr99 in CYT prevents it from interacting directly with the DH active site. The closest edge-to-edge distance between haem b and FAD is 9 Å. This distance is well within the 14-Å limit for efficient electron transfer [27] and is nearly identical to the haem-FMN distance of 9.7 Å in flavocytochrome b 2 , for which rapid IET has been observed [28] . 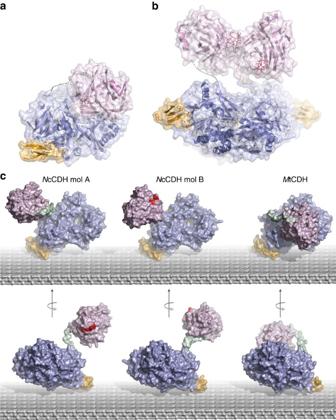Figure 1: Conformational states ofMtCDH andNcCDH. (a)MtCDH in the closed state shown as a ribbon drawing with a superimposed semitransparent surface. The missing residues 211–217 in the linker are shown as a green dotted line. Colour-coding: CYT domain (pink), DH domain (blue), CBM (orange), haemb(red), FAD (yellow). (b)NcCDH with the same colouring scheme as in (a) showing the NCS-dimer of the asymmetric unit. The missing residues 206–217 in molecule B are shown as a green dotted line. (c) The crystal structure ofNcCDH andMtCDH represented by molecular surfaces and modelled on an idealized crystalline cellulose surface. The molecules are oriented to optimize interaction of the cellulose-binding domain (orange) with the cellulose surface, and displayed in two views related by a 180° rotation to visualize the relative positions of the CYT (pink), DH (blue) and linker (green) domains. The twoNcCDH molecules A and B of the asymmetric unit have different linker conformations, revealing two unique open states. The haembgroup in the CYT domain is highlighted in red, and the entrance to the active site where the buried FAD molecule is visible (yellow) is indicated forNcCDH molecule B. For clarity, the missing residues in the linkers ofMtCDH andNcCDH have been modelled andN-linked glycans omitted. Figure 1: Conformational states of Mt CDH and Nc CDH. ( a ) Mt CDH in the closed state shown as a ribbon drawing with a superimposed semitransparent surface. The missing residues 211–217 in the linker are shown as a green dotted line. Colour-coding: CYT domain (pink), DH domain (blue), CBM (orange), haem b (red), FAD (yellow). ( b ) Nc CDH with the same colouring scheme as in ( a ) showing the NCS-dimer of the asymmetric unit. The missing residues 206–217 in molecule B are shown as a green dotted line. ( c ) The crystal structure of Nc CDH and Mt CDH represented by molecular surfaces and modelled on an idealized crystalline cellulose surface. The molecules are oriented to optimize interaction of the cellulose-binding domain (orange) with the cellulose surface, and displayed in two views related by a 180° rotation to visualize the relative positions of the CYT (pink), DH (blue) and linker (green) domains. The two Nc CDH molecules A and B of the asymmetric unit have different linker conformations, revealing two unique open states. The haem b group in the CYT domain is highlighted in red, and the entrance to the active site where the buried FAD molecule is visible (yellow) is indicated for Nc CDH molecule B. For clarity, the missing residues in the linkers of Mt CDH and Nc CDH have been modelled and N -linked glycans omitted. 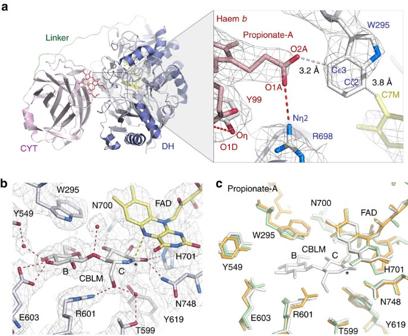Figure 2: Details of the closed state ofMtCDH. (a) Ribbon drawing (left) of the closed IET-competent state ofMtCDH showing the association of the CYT domain (pink) and the DH domain (blue). The inset (right) highlights the relative orientation of the haembin CYT (red) and the FAD (yellow) in DH (blue) with the 2F0−Fcelectron density calculated at 3.2 Å and contoured at 0.8σ. Dashed red lines represent interactions within hydrogen-bonding distance, and grey dashed lines the edge-to-edge distances for haemb-Trp295-FAD. (b) Binding of CBLM in the active site ofMtDH overlaid by a 2F0−Fcelectron density contoured at 1.3σ. The asterisk denotes the position in CBLM corresponding to the site of oxidation in cellobiose. The binding subsites are named B and C. (c) Comparison of the active site inMtCDH (orange),MtDH-CBLM (white) and ligand-freeMtDH (green). The catalytic amino acids His701 and Asn748 are positioned at there-side of the flavin. Full size image Figure 2: Details of the closed state of Mt CDH. ( a ) Ribbon drawing (left) of the closed IET-competent state of Mt CDH showing the association of the CYT domain (pink) and the DH domain (blue). The inset (right) highlights the relative orientation of the haem b in CYT (red) and the FAD (yellow) in DH (blue) with the 2 F 0 − F c electron density calculated at 3.2 Å and contoured at 0.8 σ . Dashed red lines represent interactions within hydrogen-bonding distance, and grey dashed lines the edge-to-edge distances for haem b -Trp295-FAD. ( b ) Binding of CBLM in the active site of Mt DH overlaid by a 2 F 0 − F c electron density contoured at 1.3 σ . The asterisk denotes the position in CBLM corresponding to the site of oxidation in cellobiose. The binding subsites are named B and C. ( c ) Comparison of the active site in Mt CDH (orange), Mt DH-CBLM (white) and ligand-free Mt DH (green). The catalytic amino acids His701 and Asn748 are positioned at the re -side of the flavin. Full size image We observed that crystals of native, full-length Nc CDH typically lacked interpretable density for the CYT domains. Data from one platinum-soaked crystal offered better-defined electron density for the CYT domains, which allowed us to model both Nc CDH molecules in the asymmetric unit. The overall weak density for the CYT domains suggests significant flexibility in the linker regions. The two non-crystallographically (NCS)-related molecules are present as two ‘open’ states with different conformations of the flexible linkers and different relative orientations of the CYT and DH domains ( Fig. 1 ). The haem b is fully exposed and accessible in both open-state models. The active site in CDH is accessible in the closed state The active site of CDH has two glucosyl-binding subsites for cellobiose binding, subsite B (for binding site) and C (for catalytic site) [26] , [29] . We determined the crystal structure of Mt DH in complex with the substrate analogue cellobiono-1,5-lactam (CBLM). In this complex, Trp295 acts as a platform for the non-reducing end glucosyl unit in subsite B ( Fig. 2b ). Despite differences in active site side-chain composition ( Supplementary Fig. 1 ), we observed that binding of CBLM in Mt DH is nearly identical to that previously reported for the P. chrysosporium DH co-crystal structure [29] ( Supplementary Fig. 2 ). Superimposition of the structures of Mt CDH and Mt DH-CBLM with ligand-free Mt DH revealed that only two active-site side chains differ in conformation: the indole ring of Trp295 tilts slightly ‘upwards’ with a maximum ring displacement of 1.4 Å, and Arg601 undergoes a conformational change involving 180° rotations of χ3 and χ4 on ligand binding at site B ( Fig. 2c ). Comparison of Mt CDH and Mt DH-CBLM revealed that neither the entry of propionate-A nor the binding of CBLM causes significant changes in the active site. Thus, the substrate and product can be spatially accommodated in the active site while CYT is docked onto DH in the closed state. A channel leads from the surface into the active site of the closed Mt CDH molecule. The size of this channel is sufficient ( ∼ 11 × 12 Å) to permit substrate entry and product exit while Mt CDH remains in the closed IET-competent state ( Supplementary Fig. 3 ). Analysis of the FAD–haem b interaction by mutagenesis We mutated positions in the substrate-binding region and at the CYT-DH interface ( Fig. 3 ) to investigate the validity of the closed state of Mt CDH for IET. The Mt CDH structure indicates that the haem b propionate-A in CYT interacts with four side chains in DH at the CYT-DH interface, that is, Trp295, Ser298, Met309 and Arg698, a region that we refer to as the propionate-docking site on DH. In the propionate-docking site, Trp295 performs an important role as a stacking platform for the non-reducing end glucosyl unit of the cellobiose substrate ( Fig. 2b,c ). In contrast, Ser298, Met309 and Arg698 do not interact with the substrate but with haem propionate-A ( Fig. 3 ). The variants targeting the propionate-docking site included W295A, S298Q, M309A, M309R and R698S. Another set of mutations targeted side chains in the cellobiose-binding region that could potentially affect IET, that is, Asn292, Tyr549, Tyr619 and Asn700, by generating the single mutants N292S, Y549F, Y619Q and N700S. 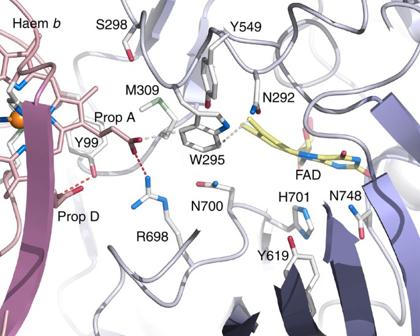Figure 3: Amino acids inMtCDH targeted for mutagenesis. Close-up of the interface between the cytochrome and dehydrogenase domains inMtCDH showing the side chains targeted for mutagenesis to evaluate the haembpropionate-A interactions in the closed state (Trp295, Ser298, Met309 and Arg698) and the substrate-binding region (Asn700, Asn292, Tyr619 and Tyr549). Figure 3: Amino acids in Mt CDH targeted for mutagenesis. Close-up of the interface between the cytochrome and dehydrogenase domains in Mt CDH showing the side chains targeted for mutagenesis to evaluate the haem b propionate-A interactions in the closed state (Trp295, Ser298, Met309 and Arg698) and the substrate-binding region (Asn700, Asn292, Tyr619 and Tyr549). Full size image Replacement of propionate-interacting residues in DH The reduction kinetics of FAD and haem b indicated that mutations that target the propionate-docking site but not substrate binding (that is, S298Q, M309A, M309R, R698S) have little impact on FAD-reduction rates but large negative effects on haem b reduction rates ( Table 1 ). A notable exception is W295A, which shows similar performance as the wild-type enzyme. At the employed high cellobiose concentration, the apparent rate of FAD reduction is not compromised by the W295A mutation. The 12% higher haem b -reduction rate of this variant is most likely due to minor structural rearrangements. The barely affected rate of this mutation demonstrates that Trp295 is not essential for IET. Table 1 FAD and haem b reduction kinetics of Mt CDH wild type and variants. Full size table The side chain of Ser298 packs against the haem b methyl group (attached to pyrrole ring A), adjacent to propionate-A ( Fig. 3 ). Replacing Ser298 with glutamine leads to a minor decrease of 18% in the FAD-reduction rate, while the haem b reduction rate decreases drastically by 88% ( Table 1 ). The decrease in haem b k obs for S298Q can be rationalized by steric clashes between the longer glutamine side chain and haem pyrrole A (and with Gln175) in CYT that push propionate-A out from the propionate-docking site on DH. In the wild-type enzyme, Met309 forms van der Waals interactions with the aliphatic carbons of the propionate-A side chain and Tyr99 in CYT, as well as with Trp295, Arg698, Asn700 and the FAD 8-methyl group in DH ( Fig. 3 ). Most, if not all, of these interactions would be eliminated in the M309A mutant, which also exhibits a drastic decrease in the haem b reduction rate. Thus, Met309 is important for CYT-DH association, but interpretation of the effects of this mutation is complicated by the threefold reduction in the FAD-reduction rate, which indicates that the mutation has effects beyond the precise association of the functional domains. Another replacement at this position, M309R, maintains the aforementioned interactions with an unperturbed FAD-reduction rate while selectively interfering with propionate-A docking. The loss of IET in this mutant is attributable to the longer arginine side chain, which either pushes CYT away from the propionate-docking site on DH or locks the propionate-A carboxyl group in an ionic interaction. The guanidium group of Arg698 interacts directly with propionate-A, and replacing this side chain with serine abolishes haem b reduction without affecting the FAD reduction rate, which is consistent with the observed structure of the closed state of Mt CDH. Replacement of residues in the substrate-binding region The side chain of Asn292 is positioned in subsite B, close to Trp295, but does not interact with either CYT or the haem b group ( Fig. 3 ). The FAD-reduction rate is increased by 20% for the N292S mutant at the high concentration of cellobiose (25 mM), with a proportional increase in the rate of haem b reduction ( Table 1 ). Asn292 has no significant direct effect on the CYT-DH association or IET, which is also in agreement with the closed Mt CDH structure. Another residue at the DH active-site entrance is Tyr549 ( Fig. 3 ), which is located in the channel that runs across the CYT-DH interface. Here Tyr549 makes no direct contact with either the CYT domain, haem b propionates, or substrate and is therefore not expected to affect either the CYT-DH association or IET. The unperturbed FAD and haem b reduction rates of Y549F confirm that the Tyr549 hydroxyl group is not important for IET. The side chain of Tyr619 is located in subsite C in DH, where it likely stabilizes the transition state during cellobiose oxidation [29] . We observed a 2-fold decrease in the k obs values for both FAD and haem b reduction for Y619Q. The pronounced decrease in the FAD-reduction rate indicates that this variant is catalytically defective, which suggests that Tyr619 has functions other than promoting IET. The side chain of Asn700 packs against the dimethyl benzene nucleus of FAD, where it can form a hydrogen bond with the O3 hydroxyl of the reducing-end glucosyl of cellobiose in subsite C ( Figs 2b and 3 ) and with Arg698. The variant N700S displays a 1.3-fold increase in the FAD-reduction rate and a disproportionally higher 1.8-fold increase in the haem b reduction rate. The selective improvement in the IET rate may be due to an increase in the volume of the propionate-docking site caused by the substitution with the smaller serine residue, which may allow Arg698 to move closer to FAD, and consequently, bring propionate-A closer to the flavin. Solution structures of CDH We used small-angle X-ray scattering (SAXS) analysis to investigate the conformational space of CDH in solution using the ensemble-optimization method (EOM), which employs a genetic algorithm for the selection of conformers from pools of randomly generated models [30] , [31] . SAXS was performed on glycosylated and deglycosylated Mt CDH and Nc CDH in the absence and presence of bound inhibitor (CBLM). Our results demonstrated that all Mt CDH and Nc CDH samples contain similar subsets of conformers in solution ( Supplementary Figs 4 and 5 ). The conformer most similar to the closed state in the crystal structure of Mt CDH is present in all samples (deglycosylated Mt CDH cluster 5, deglycosylated Mt CDH/CBLM cluster 3, glycosylated Mt CDH cluster 1 and glycosylated Mt CDH/CBLM cluster 4 in Supplementary Fig. 4 ). In the presence of inhibitor, the ensemble of glycosylated Mt CDH exhibits fewer conformers in solution, with an open state resembling molecule A in the crystal structure of Nc CDH as the most populated species (45%) and a closed state resembling the Mt CDH crystal structure as the second most populated conformer (27%). Conformers resembling the closed state are also present in all Nc CDH samples (deglycosylated Nc CDH cluster 8, deglycosylated Nc CDH/CBLM cluster 7, glycosylated Nc CDH cluster 2 and 3, and glycosylated Nc CDH/CBLM cluster 1 and 4 in Supplementary Fig. 5 ). As with Mt CDH, glycosylated Nc CDH exhibits an ensemble with fewer conformational clusters in the presence of inhibitor. We also confirmed that glycosylated and deglycosylated Mt CDH and Nc CDH were present in solution as monomers by performing chemical cross-linking, size-exclusion chromatography and native PAGE (data not shown). Crystal structure of Nc LPMO 9F Nc LPMO 9F primarily attacks crystalline cellulose and promotes, in combination with cellulases, faster and more complete surface degradation [32] . The structure of Nc LPMO 9F demonstrates that this LPMO shares the essential features of fungal LPMOs, including a β-sandwich fold and a catalytic surface-exposed copper centre ( Fig. 4a ) in which the copper is coordinated by the ligands His1, His72 and Tyr157 ( Fig. 4b,c ). Fungal LPMOs are typically post-translationally modified by protein glycosylation and methylation at the N-terminal histidine (the function of this methylation is unknown). We determined that Nc LPMO 9F is expressed in Pichia pastoris as a 214-residue non-glycosylated protein. As observed for the fungal LPMO GH61D from Phanerochaete chrysosporium [33] , the N-terminal histidine in Nc LPMO 9F is not methylated, in contrast to the methylation of other N. crassa LPMOs expressed using the natural fungal host [15] , [23] . Both NCS molecules in the NcLPMO 9F crystal have copper ligated by four protein atoms in tetrahedral coordination and exhibit distorted octahedral coordination of the copper with mer -[MA 3 B 3 ] geometry together with external ligands ( Fig. 4b,c ; Supplementary Fig. 6 ). In molecule A, two water molecules, one axial and one equatorial, satisfy the octahedral sphere ( Fig. 4b ; Supplementary Fig. 6a ). In molecule B, both water molecules are replaced by the carboxylate oxygen atoms of Asp33 from molecule A ( Fig. 4c ; Supplementary Fig. 6b ), which is similar to the coordination sphere observed in Streptomyces coelicolor Sc LPMO 10B where two oxygen atoms in an acetate molecule occupy the fourth equatorial and axial position on the solvent-facing side of Cu(II) [34] . These observations emphasize the possibility of the 4-coordinate Cu(II) in Nc LPMO 9F to accept one axial, and possibly also a fourth equatorial ligand (water or other). 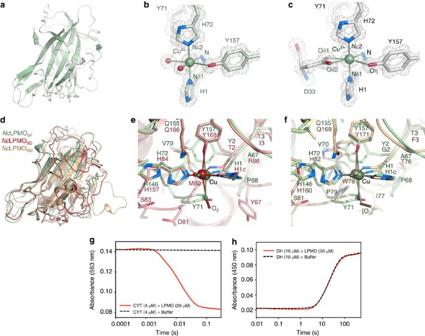Figure 4: Structure ofNcLPMO9Fand interaction withNcCYT. (a) Overall structure ofNcLPMO9F. (b) Distorted octahedral coordination for the copper inNcLPMO9Fmolecule A (green). The three nitrogen ligands provided by His1 and His72 are referred to as thehistidine brace10. Coordination is satisfied by two water ligands (seeSupplementary Fig. 6for details). Overlay with 2F0−Fcelectron density (1.5σ). (c) Cu(II) coordination inNcLPMO9Fmolecule B (white). Octahedral coordination is satisfied by replacing the water ligands in (b) by two oxygen atoms from Asp33 (green) in the NCS-related A molecule. (d) Structural overlay ofN. crassaLPMO9F(green) withN. crassaPMO-2 (red; PDB code 4EIR23) and PMO-3 (beige; PDB code 4EIS23). (e) Comparison of the copper centres inNcLPMO9F(green) and PMO-2. (f) Comparison of the copper centres inNcLPMO9F(green) and PMO-3. The residue H1crepresents a methylated N-terminal histidine. (g) Interaction betweenNcCYT andNcLPMO9Fdisplayed as an averaged kinetic trace (full line). The calculated haem re-oxidation rate from five repeated experiments (kobs) is 67.2±2.3 s–1. For comparison, the haem re-oxidation by oxygen is shown as a dashed line. (h) The re-oxidation rates of the FAD cofactor of theNcCDH dehydrogenase domain (10 μM) remains unchanged in the presence (0.0442 +/−0.0003, s–1) and absence (0.0444 +/− 0.0006, s–1) of 50 μM LPMO, showing that no reduction of theNcLPMO9FCu(II) centre takes place. The observed low rates are the result of a re-oxidation reaction with dissolved oxygen in the buffer. Figure 4: Structure of Nc LPMO 9F and interaction with Nc CYT. ( a ) Overall structure of Nc LPMO 9F . ( b ) Distorted octahedral coordination for the copper in Nc LPMO 9F molecule A (green). The three nitrogen ligands provided by His1 and His72 are referred to as the histidine brace [10] . Coordination is satisfied by two water ligands (see Supplementary Fig. 6 for details). Overlay with 2 F 0 − F c electron density (1.5 σ ). ( c ) Cu(II) coordination in Nc LPMO 9F molecule B (white). Octahedral coordination is satisfied by replacing the water ligands in ( b ) by two oxygen atoms from Asp33 (green) in the NCS-related A molecule. ( d ) Structural overlay of N. crassa LPMO 9F (green) with N. crassa PMO-2 (red; PDB code 4EIR [23] ) and PMO-3 (beige; PDB code 4EIS [23] ). ( e ) Comparison of the copper centres in Nc LPMO 9F (green) and PMO-2. ( f ) Comparison of the copper centres in Nc LPMO 9F (green) and PMO-3. The residue H1 c represents a methylated N-terminal histidine. ( g ) Interaction between Nc CYT and Nc LPMO 9F displayed as an averaged kinetic trace (full line). The calculated haem re-oxidation rate from five repeated experiments ( k obs ) is 67.2±2.3 s –1 . For comparison, the haem re-oxidation by oxygen is shown as a dashed line. ( h ) The re-oxidation rates of the FAD cofactor of the Nc CDH dehydrogenase domain (10 μM) remains unchanged in the presence (0.0442 +/−0.0003, s –1 ) and absence (0.0444 +/− 0.0006, s –1 ) of 50 μM LPMO, showing that no reduction of the Nc LPMO 9F Cu(II) centre takes place. The observed low rates are the result of a re-oxidation reaction with dissolved oxygen in the buffer. Full size image The crystal structures of N. crassa Nc LPMO 9D (PMO-2; PDB code 4EIR [23] ; NCU01050; UniProt Q1K8B6) and Nc LPMO 9M (PMO-3; PDB code 4EIS [23] ; NCU07898; UniProt Q7SA19) have been determined at high resolution. While the overall fold of Nc LPMO 9F is very similar to those of Nc LPMO 9D (r.m.s.d. 1.45 Å for 205 Cα positions) and Nc LPMO 9M (r.m.s.d. 1.35 Å for 189 Cα positions), significant conformational changes are apparent in loop regions, including loops flanking the copper-binding site ( Fig. 4d ). In contrast to Nc LPMO 9F , Nc LPMO 9D and Nc LPMO 9M are glycosylated and have a methylated N-terminal histidine ( Fig. 4e,f ). Furthermore, the axial ligand occupied by water or Asp33 Oδ1 in Nc LPMO 9F ( Fig. 4b,c ; Supplementary Fig. 6 ) is modelled as superoxide and peroxide in Nc LPMO 9D ( Fig. 4e ) and Nc LPMO 9M ( Fig. 4f ), respectively. Beyond the copper ligands, the amino-acid context differs in Nc LPMO 9F compared with Nc LPMO 9D and Nc LPMO 9M ( Supplementary Fig. 7 ). Nc CYT but not Nc DH transfers electrons to Nc LPMO 9F Next we performed rapid-kinetics experiments to confirm that direct ET occurs between Nc CYT and Nc LPMO 9F ( Fig. 4g ). We observed very rapid Nc CYT-to- Nc LPMO 9F ET with a haem b - k obs value of 67.2±2.3 s –1 . The re-oxidation rate of Nc CYT by oxygen was 100,000-fold slower (0.0007, s −1 ) than the rate for Nc CYT-to- Nc LPMO 9F ET, making the oxygen reaction negligible. To further rule out reduction of the Nc LPMO 9F copper centre by the FAD cofactor in the Nc CDH dehydrogenase, we performed a second stopped-flow experiment, which demonstrated conclusively that the Nc DH domain alone is unable to reduce Cu(II) in Nc LPMO 9F ( Fig. 4h ). Our results demonstrate unequivocally that, in the N. crassa CDH IIA-LPMO 9F pair, the reduced haem b alone acts as the reductant of the Nc LPMO 9F copper centre in vitro . The high ET rate observed in the study provides compelling evidence for LPMO as a physiologically relevant electron acceptor for the haem b cytochrome. To test the interaction of the Nc CDH- Nc LPMO 9F pair, we performed automatic high ambiguity-driven biomolecular docking ( HADDOCK ). The program consistently returned interaction models where the haem b propionate-A was docked close to the copper in Nc LPMO 9F . The docking of solvated proteins does not consider the constrained accessibility of the copper site in cellulose-bound LPMO; however, in solution and when freely accessible, the copper site appears to be a favourable docking site for the haem b propionate ( Supplementary Fig. 8 ). Because no information concerning the precise copper-haem coordination geometry had been provided to the program, the precise details of the automatically generated CYT-LPMO interaction models cannot be evaluated; however, the interaction energies are favourable. The crystal and solution structures of two closely related class-II CDHs revealed pronounced flexibility of the linker between the CYT and DH domains to allow the efficient association of the haem b with both the FAD electron donor (closed state) and external protein electron acceptors such as LPMO (open states). Using SAXS, we demonstrated that the conformers observed in the crystal structures are also present in solution and performed comprehensive mapping of accessible CDH conformers, including the closed state and a range of partially closed and open states. Moreover, our data demonstrate that similar CDH conformers are possible for glycosylated and deglycosylated samples and that the presence of an inhibitor reduces the number of accessible conformers in solution. The crystal structure of the closed state of Mt CDH offers a favourable association mode between the CYT and DH domains to permit efficient IET. The validity of the closed state is further emphasized by the drastically decreased IET rates of Mt CDH variants in which the interactions between haem b propionate-A and DH at the CYT-DH interface have been disabled. Whereas the IET rates were diminished for mutations targeting the propionate-docking site, we observed no systematic effects on IET rates for the mutations targeting side chains in the substrate-binding region occupying the space between the flavin and propionate-A. These results allow us to assign a fundamental role to the haem b propionate-A in the IET mechanism. Haem propionate groups actively participate in ET events. For example, the use of mixed quantum mechanical/molecular mechanics calculations has provided direct evidence for the active involvement of haem-propionate groups in the ET pathway of ascorbate peroxidase and di-haem- c cytochrome c peroxidase [35] . Our results, together with the low sequence conservation between ascomycete and basidiomycete CDHs (of the mutated residues, only Tyr619, Asn700 and Tyr549 are conserved in Pc CDH; Supplementary Fig. 1 ), emphasize that efficient IET does not depend intimately on any one specific type of side chain but on the ability of CYT to associate with DH in a manner in which the relative position and distance between the haem propionate and FAD ensure IET. In contrast to the intracellular enzyme flavocytochrome b 2 , CDH is an extracellular flavocytochrome. A variety of two-electron acceptors are generated during lignocellulose decomposition, for example, lignin-derived quinone compounds that would react rapidly with reduced FAD. How is specific FAD-haem b IET ensured in this extracellular environment containing electron scavengers? If CYT docks with DH before substrate binding and remains docked during IET (and possibly after product departure), the IET path would be shielded both by the CYT-DH interface and by the bound product, thus preventing electron scavengers from accessing the reduced FAD before the haem b is reduced and CYT is released. Indeed, various free one-electron acceptors such as Fe(III) and Cu(II) complexes are present in wood and could scavenge electrons from reduced CYT upon release from DH. The surfaces near the channel entrance in Mt CDH are rich in negatively charged residues that do not participate in complex formation ( Supplementary Fig. 9a ). It is tempting to speculate that their function may be to guard the entrance to allow carbohydrates to enter and exit, while metal ions are chelated and negatively charged molecular species are repelled. Overall, Nc CDH has fewer negative surface residues but displays a similar trend of negative charges clustering near the channel entrance ( Supplementary Fig. 9b ). In this work, we demonstrate that only the CYT haem b of Nc CDH can transfer electrons to Nc LPMO 9F and that DH alone is not an electron donor for LPMO. We expect this ET to manifest as a physical but not necessarily strong or long-lived protein complex. On the basis of global sequence conservation within the LPMO family, a conserved surface patch centred on 218 Pro-Gly-Pro 220 (numbering of Nc PMO 9M ) has been suggested as an interaction site for CDH [23] . The patch is positioned 21 Å from the copper centre, and its involvement assumes long-range electron tunnelling through the protein to reach the site of reduction. Such a scenario seems mechanistically reasonable for LPMO where, during catalysis, the copper-site is expected to be oriented towards the cellulose surface and therefore is inaccessible for a direct interaction with the redox centre in CYT. It is therefore surprising to find no conserved complementary surfaces on CYT. Rather, the haem b propionate-A, which protrudes from the CYT surface and restricts surface complementarity between CDH and LPMO at the proposed interaction site, is the only absolutely conserved surface feature among different CDHs. Because CDH has to form a CYT–DH IET complex and has been observed to transfer electrons to a variety of LPMOs with different surface properties and even from different organisms, it is not surprising that the interacting interfaces display an overall low degree of surface complementarity. The results from ambiguity-driven biomolecular protein-protein docking suggest an alternative binding mode for LPMO when not bound to cellulose where the copper-binding surface provides the most favourable interaction site for CYT. However, it is not possible to evaluate the significance of such an interaction by automated molecular docking alone and mutational studies are needed to elucidate the in vivo interaction site. At present, two principal LPMO mechanisms for glycosidic bond cleavage have been proposed. The first mechanism involves sequential ET [17] , in which an initial electron reduces Cu(II) to Cu(I), leading to the formation of a Cu(II)-superoxo complex. A second electron is required after hydrogen abstraction from the substrate to cleave the O-O bond in the Cu(II)-hydroperoxo species, releasing water and generating a Cu(II)-oxo radical that couples with the substrate radical and leads to the hydroxylation of the substrate. The second mechanism, which was suggested based on quantum mechanical calculations, proposes C-H oxidation by a Cu(II)-oxyl mechanism [24] and argues that a Cu(II)–oxyl complex is more reactive than the Cu(II)–superoxo complex and that the Cu(II)–oxyl species has a lower overall activation barrier than the Cu(II)–superoxo species. This model hypothesizes two electron transfer events in series before LPMO reacts with cellulose. In both cases, hydroxylation at C1 or C4 destabilizes the glycosidic bond, and an elimination reaction leads to bond cleavage. Both models are compatible with one-electron transfer from CYT to LPMO, but the precise structural and mechanistic details of the CYT-LPMO interaction need further investigation. In this work, we have presented for the first time the structural basis for electron transfer between FAD and haem b in CDH, and shown that the cytochrome alone is responsible for rapid electron transfer to LPMO. Our results provide the structural foundation towards a full molecular understanding of the role of the CDH-LPMO system in oxidative cellulose degradation by fungi. Enzyme production Cloning of all genes has been reported: Myriococcum thermophilum CDH [36] ( Mt CDH IIA; gene cdh ; UniProt A9XK88; the DH domain belongs to CAZy family AA3_1 and the CYT domain to CAZy family AA8 (ref. 37 )), Neurospora crassa CDH IIA [21] ( Nc CDH; gene cdh-1 ; locus tag NCU00206; UniProt Q7RXM0; the DH domain belongs to CAZy family AA3_1 and the CYT domain to CAZy family AA8 (ref. 37 )) and Neurospora crassa LPMO Nc LPMO 9F (ref. 38 ) (gene gh61-6 ; locus tag NCU03328; UniProt Q1K4Q1; CAZy family AA9). The Mt CDH variants were generated by a two-step mutagenesis approach using PCR and Dpn I. The replacements included N292S, W295A, S298Q, M309A, M309R, Y549F, Y619Q, R698S and N700S. The mutations were confirmed by sequencing. Fed-batch fermentations of Pichia pastoris X-33 transformants were performed in a 7-litre bioreactor (MBR, Switzerland) with 3 litre starting volume following the Pichia Fermentation Process Guidelines of Invitrogen. After depletion of glycerol in the batch medium a 12-h fed-batch phase was started with a constant feed of 50% glycerol containing 12 ml l –1 PTM 1 trace salts to increase biomass. For induction the feed was switched to pure methanol containing 12 ml l –1 PTM 1 trace salts and the cultivation temperature was reduced from 30 to 25 °C. At the time the culture fully adapted to methanol the feed rate was automatically adjusted to keep the dissolved oxygen saturation constant at 4% at a constant air supply of 6 l min –1 and a stirrer tip speed of 2.95 m s –1 . Samples were taken regularly and wet biomass, protein concentration and enzyme activity were measured. Fermentation broths were harvested by centrifugation before the expression of the targeted enzymes stagnated. Wild type and mutant CDHs were expressed in concentrations from 50 to 400 mg l –1 , and the protein concentration of Nc LPMO 9F in the culture supernatant was 750 mg l –1 . Additional details have been reported elsewhere [36] , [38] , [39] , [40] . Enzyme purification Nc DH, Nc CYT, Nc CDH, Mt DH and Mt CDH variants were purified by a two-step chromatographic procedure starting with hydrophobic interaction chromatography using PHE-Sepharose FF (all chromatographic equipment and materials from GE Healthcare Biosciences). Proteins were applied in a 50 mM sodium acetate buffer (pH 5.5) containing 20% ammonium sulfate (saturation) and eluted by a linear gradient against the same buffer without ammonium sulfate. Fractions containing the target enzyme were pooled and diafiltered with a 50 mM sodium acetate buffer (pH 5.5) using a hollow fibre cross-flow module (Microza UF module SLP-1053, 10 kDa cut-off, Pall Corporation). Concentrated CDH pools were applied to a column packed with Source 15Q material equilibrated with 50 mM sodium acetate buffer (pH 5.5) and eluted within a linear salt gradient from 0 to 1 M NaCl within 10 column volumes. Nc LPMO 9F was purified by a three-step chromatographic procedure starting with hydrophobic interaction chromatography using PHE-Sepharose FF. The protein was loaded in 25 mM sodium acetate buffer (pH 5.0) containing 30% ammonium sulfate (saturation), and eluted by a linear gradient. Fractions containing the enzyme were pooled and diafiltered with a 20 mM Tris-HCl buffer (pH 8.0) using a hollow fibre cross-flow module. After reaching a conductivity below 1.4 mS cm –1 the pool was applied to a column packed with Source 15Q. The flow-through contained Nc LPMO 9F and was concentrated and further purified with size-exclusion chromatography using a Superdex 75 column equilibrated with 20 mM Tris-HCl buffer (pH 8.0). Fractions containing pure Nc LPMO 9F were pooled, concentrated to a final concentration of 6.5 mg ml –1 and stored at 4 °C. Deglycosylation and proteolytic cleavage of CDHs The purified CDHs were treated at 30 °C for 18 h with 3,200 U ml –1 α-1,2/3-mannosidase and 50,000 U ml –1 endoglycosidase H f (New England Biolabs, Ipswich, MA, USA) in 50 mM sodium acetate buffer (pH 5.5) containing 5 mM ZnCl 2 to obtain 10 mg ml –1 deglycosylated enzyme. To remove the glycosidases, column chromatography with Source 15Q was repeated as described above and the fractions containing pure CDH were pooled, diafiltered to 50 mM sodium acetate buffer (pH 5.5) and stored at 4 °C. Proteolytic cleavage in the linker of CDH was performed to obtain the individual DH and CYT domains. To this end, 40 μl of papain (10 mg ml –1 ) was incubated at 25 °C for 1 h with 100 μl of activation buffer containing 2 mM EDTA and 2 mM dithiothreitol in 100 mM sodium phosphate (pH 7.0). CDH (final concentration 10 mg ml –1 ) was digested in a reaction mix containing 140 μl per ml of the activated papain solution and 1 M sodium acetate (pH 5.0) at 25 °C for 4 h. The domains were separated from the residual intact CDH by column chromatography using a strong anion exchanger (Mono Q). The sample was diafiltered to 20 mM Tris-HCl (pH 8.0), loaded on the column and eluted by a linear NaCl gradient. Fractions containing the dehydrogenase and the cytochrome domain were pooled, concentrated and stored at 4 °C for further use. Kinetic characterization of Mt CDH wild type and variants Pre-steady-state measurements were carried out in a stopped-flow spectrophotometer (Applied Photophysics SX 20, Leatherhead, UK) at 30 °C. The concentration of enzymes was determined by their molar absorption coefficients ( Nc CDH ɛ 420 =100 mM –1 cm –1 , Nc DH ɛ 450 =11.3 mM –1 cm –1 , Nc LPMO 9F ɛ 280 =46.9 mM –1 cm –1 ). The FAD and haem b reduction rates in CDH were measured at 449 and 563 nm, respectively, by reducing 5 μM CDH with 25 mM cellobiose (final concentrations) in 50 mM sodium citrate buffer pH 5.0. Electron transfer Nc CYT– Nc LPMO 9F and Nc DH– Nc LPMO 9F The same technique was used for measuring the ET between Nc CYT or Nc DH and Nc LPMO 9F . Nc CYT was partially reduced with sodium dithionite (15 mM stock solution) by following the spectra in a diode array photometer. By partial reduction, excess of reductant was prevented. The 50% reduced Nc CYT was immediately transferred to a stopped-flow spectrophotometer and mixed with Nc LPMO 9F in single mode. Re-oxidation of the α-band of Nc CYT haem b was recorded at 563 nm. Concentrations in the cell were 4 μM reduced Nc CYT and 20 μM Nc LPMO 9F in 50 mM sodium citrate buffer pH 5.0. The observed rates were fitted to a single exponential function. Reduction and re-oxidation of the FAD cofactor in DH was followed at 450 nm. Experiments were performed in sequential mode by mixing 40 μM Nc DH with 100 μM cellobiose to reduce the enzyme. The reaction was held in an ageing loop for 75 s until ∼ 10% of the Nc DH was re-oxidized. The partly re-oxidized Nc DH was shot against buffer or Nc LPMO 9F . Final concentrations in the measuring cell were 10 μM Nc DH and 50 μM Nc LPMO 9F . The rates were calculated from an exponential fit. Crystallization, structure determination and model refinement Data collection and refinement statistics are given in Table 2 . All protein crystallization was performed using the sitting-drop vapour diffusion method at room temperature. Image processing and data scaling were performed with the XDS package [41] . When applicable, molecular replacement (MR) was performed using PHASER [42] as implemented in the PHENIX suite [43] , and unless otherwise stated experimental phasing was performed with autoSHARP [44] . Manual model building and correction was performed with the programs O [45] and COOT [46] . Experimental details for each protein are given below. For models refined at lower resolution, the resolution cutoff for refinement was guided by the CC (1/2) values, that is, the percentage of correlation between intensities from random half data sets [47] . Table 2 Data collection, phasing and refinement statistics. Full size table MtCYT (MtCDH cytochrome domain) . Crystals of deglycosylated Mt CYT were obtained by mixing equal volumes of protein solution (21 mg ml –1 in 20 mM HEPES pH 7.5) and a solution containing 0.1 M Tris-HCl (pH 8.4), 0.2 M MgCl 2 , 30% (w/v) polyethylene glycol 4,000. The crystals belong to space group P 2 1 with two molecules in the asymmetric unit. A model for molecular replacement (MR) was generated automatically using the BALBES server [48] . MR calculations were performed with PHASER , and a model was traced and built automatically using data to 1.4 Å resolution with the warpNtrace function in ARP/wARP [49] . The model was refined at 1.4 Å resolution with PHENIX , using the maximum-likelihood target and including refinement of coordinates, real-space refinement and refinement of individual anisotropic temperature factors ( Table 2 ; Supplementary Fig. 10a ). The refined model contains: two protein chains, A and B, each composed of residues 1–208 (corresponding to residues 22–229 in UniProt A9XK88); one type- b protoheme IX group per protein chain; protein glycosylation (one N -acetyl glucosamine, NAG, residue attached to Asn119, and four O -linked mannose residues attached to Ser195, Thr197, Thr204 and Thr206, respectively, per protein chain); one magnesium ion bound to protein chain A and two magnesium ions to chain B; and 350 water molecules. MtDH (MtCDH dehydrogenase domain) . Non-deglycosylated Mt DH crystallized from mixing equal volumes of a solution containing 0.1 M sodium acetate (pH 4.6), 0.1 M CdCl 2 , 18% (w/v) polyethylene glycol monomethyl ether 550 with protein (58 mg ml –1 in 20 mM HEPES pH 7.5). The crystals belong to space group P 6 3 with one molecule in the asymmetric unit. Cryo protection was performed by equilibration in a solution containing the crystallization liquor, but with 30% (w/v) polyethylene glycol monomethyl ether 550. Data were collected on a native crystal, as well as two heavy-atom derivatives, lead acetate and mercury acetate. The heavy atoms were added as powder to the cryo-protection solution and the crystals left to equilibrate in the presence of heavy atom for 1 min before being vitrified in liquid nitrogen. For the complex of Mt DH with the inhibitor 5-amino-5-deoxy-cellobiono-1,5-lactam (CBLM) a crystal was used that resulted from equal volumes of 58 mg ml –1 protein in 20 mM HEPES pH 7.5 and 0.1 M sodium acetate (pH 4.6), 0.1 M CdCl 2 , 15% (w/v) polyethylene glycol monomethyl ether 2000. The crystal was equilibrated in a solution containing 0.1 M sodium acetate (pH 4.6), 0.1 M CdCl 2 , 30% (w/v) polyethylene glycol monomethyl ether 2000 and 2 mM cellobionolactam inhibitor. The Mt DH structure was determined using multiple isomorphous replacement with anomalous scattering (MIRAS) with lead acetate and mercury acetate using autoSHARP [44] . SHELXD [50] in autoSHARP was used to locate the heavy-atom positions, and SHARP [44] to refine heavy-atom positions and calculate phases. Density modification using a solvent content of 66% was performed with SOLOMON in autoSHARP and DM in the CCP4 suite [51] . The final MIRAS phases to 3 Å were of high quality and during the process of iterative model building and refinement, averaged structure factors from the derivatives where the heavy-atom contribution had been removed ( F av ) were used together with Hendrickson–Lattman coefficients to allow phase combination of experimental MIRAS phases with partial model phases ( F c ) in REFMAC5 [52] to improve refinement, phases and 2F 0 –F c electron density quality. The structure of the Mt DH–CBLM complex was determined by MR with PHASER using the Mt DH model as search probe. The software PHENIX was used to refine the Mt DH and Mt DH-CBLM models at 2.7 and 2.4 Å resolution, respectively ( Table 2 ; Supplementary Fig. 10b,c ). Refinement incorporated the maximum-likelihood target, refinement of coordinates, real-space refinement, refinement of individual isotropic temperature factors and translation-libration-screw (TLS) refinement using TLS groups derived by the PHENIX software (five groups for Mt DH and six groups for Mt DH–CBLM). The refined Mt DH model contains: one protein chain (A) composed of residues 223–807 (corresponding to residues 244–828 in UniProt A9XK88); one non-covalently bound FAD molecule; protein glycosylation (two NAG residues attached to Asn400, two NAG residues at Asn437, and one NAG at Asn516); 9 cadmium ions; and no water molecules. The resulting Mt DH-CBLM model contains: one protein chain (A) composed of residues 223–807; one non-covalently bound FAD molecule; protein glycosylation (two NAG residues attached to Asn400 and two NAG residues at Asn437); one CBLM molecule; two cadmium ions; and 182 water molecules. MtCDH . Deglycosylated Mt CDH was crystallized from mixing equal volumes of 0.1 M MES-OH (pH 6.5), 0.1 M ammonium sulfate, 0.4 M sodium formate, 30% (w/v) polyethylene glycol monomethyl ether 5,000 with protein (84 mg ml –1 in 20 mM sodium acetate pH 5.5). The crystals were in point group 422, with one molecule in the asymmetric unit. The space group was deduced at the structure determination stage. The individual Mt CYT and Mt DH domains, refined at 1.4 Å and 3.0 Å resolution, respectively, and Mt CDH data (4.5–15 Å) were used for MR calculations using PHASER . All possible PG422 enantiomorphs were tested, returning a clear solution only in space group P 4 3 2 1 2. The Mt CDH model was refined against the maximum-likelihood target in PHENIX at 3.2 Å resolution ( Table 2 ; Supplementary Fig. 11a ) using a refinement protocol including XYZ coordinate refinement, refinement of grouped isotropic temperature factors (two groups per residue). The refined Mt CDH model contains one protein chain (A) composed of residues 1–807 (corresponding to residues 22–828 in UniProt A9XK88; 1–21 belong to the signal peptide) with residues 211–217 of the linker missing; one type- b protoheme IX group; one non-covalently bound FAD molecule; and protein glycosylation (one NAG residue attached to Asn400, Asn437, Asn516 and Asn678; one mannose residue attached to Ser195, Thr197, Thr204, Thr206 and Thr226). NcCDH . Deglycosylated Nc CDH was crystallized from mixing equal volumes of 0.1 M MES-OH (pH 6.5), 1.5 M magnesium sulfate, 0.02 M lithium sulfate with protein (36 mg ml –1 in 20 mM sodium acetate pH 5.5). Crystals were equilibrated in the crystallization solution supplemented with 50% saturated lithium sulfate before being vitrified in liquid nitrogen. The crystals were in space group P 2 1 2 1 2 1 with two molecules in the asymmetric unit. The platinum derivative was produced by adding K 2 Pt(CN)4 powder to a drop containing the crystal in its mother liquor. Initial phasing was performed using Pt-SAD in autoSHARP . Phases were improved by density modification with SOLOMON using a solvent content of 61.3% to 2.9 Å resolution. To facilitate model building, the Mt CYT and Mt DH domains were placed in the Nc CDH unit cell using MR calculations with PHASER . Model re-building was guided by MR- and SAD-phased electron-density maps. Both Nc CDH molecules in the asymmetric unit are in the open conformation with dissociated CYT and DH domains. The inherent flexibility of the linker connecting the CYT and DH domains resulted in different NCS symmetry for the CYT and DH domain pairs in the asymmetric unit, and partly disordered linker regions. The Nc CDH model was refined using the maximum-likelihood target in PHENIX at 2.9 Å resolution ( Table 2 ; Supplementary Fig. 11b ) using a refinement protocol including XYZ coordinate refinement, refinement of individual isotropic temperature factors and TLS refinement (six groups). The refined model contains two protein chains (A and B) composed of residues 2–806 (corresponding to residues 25–829 in UniProt Q7RXM0; 1–23 belongs to the signal peptide) with residues 206–217 in the linker missing in protein chain B; one type- b protoheme IX group and one non-covalently bound FAD molecule per protein chain; protein glycosylation (Asn119, Asn278, Asn400, Asn471, Asn515, Asn541 and Asn555 each have one N -linked NAG residue); one mannose residue attached to Thr222 and Thr226; and 10 platinum atoms bound per protein chain. Nc LPMO 9F . Nc LPMO 9F is natively non-glycosylated and contains one copper centre. The copper content of purified Nc LPMO 9F was analysed by inductively coupled plasma atomic emission spectroscopy, ICP-AES, and sector field inductively coupled plasma mass spectroscopy, ICP-SMS (ALS Scandinavia AB). Crystals of Nc LPMO 9F were produced by mixing 0.1 μl of protein (30 mg ml –1 in 50 mM Tris pH 8.0) with 0.2 μl of reservoir solution containing 0.2 M ammonium nitrate and 20% (w/v) polyethylene glycol 3350. The crystals belong to space group P 2 1 2 1 2 with two molecules in the asymmetric unit. Structure determination was performed by taking advantage of the copper centre for Cu-SAD using the AutoSol and AutoBuild modules in PHENIX . The best SAD solution had an estimated map CC × 100 of 29.0 +/− 28.3. Density modification and model building were performed iteratively by RESOLVE [53] using a default solvent content of 50%, yielding a model with an R factor of 0.28 and a correlation of local RMS density of 0.75. The Nc LPMO 9F model was refined using data at 1.1 Å resolution ( Table 2 ; Supplementary Fig. 11c ) with PHENIX , using the maximum-likelihood target and including refinement of XYZ coordinates, real-space refinement, refinement of individual anisotropic temperature factors, and riding hydrogen atoms. The refined Nc LPMO 9F model contains two protein chains (A and B) each composed of residues 1–214 (corresponding to residues 18–231 in UniProt Q1K4Q1; 1–17 constitutes a signal peptide); one copper per protein chain; one nitrate molecule in chain B, and 838 water molecules. Modelling of Nc CDH- Nc LPMO 9F was performed by manual docking of Nc CDH CYT such that the haem b propionate-A carboxyl group superimposed with that of the copper-coordinating Asp33 in NCS molecule A of Nc LPMO 9F . SAXS data collection and analysis Samples of deglycosylated and glycosylated Mt CDH and Nc CDH were prepared at the concentrations 1, 2.5 and 10 mg ml –1 in 50 mM sodium acetate (pH 4.5), and in the absence or presence of 1 mM CBLM. Data were collected through mail-in-SAXS on the 12.3.1 SIBYLS beamline at the Advanced Light Source, Lawrence Berkeley National Laboratory [54] , [55] , and at the MAX II SAXS beamline I 911-SAXS [56] at MAX IV Laboratory, Lund, Sweden. Data were processed using PRIMUS [57] in the ATSAS suite [31] . The ensemble optimization modelling method [30] , [31] was used to generate the most populated clusters of conformers in an ensemble that best fits the scattering data. The crystal structures of CYT and DH were input as domains and 10,000 models with different domain orientations and automatically modelled linkers were generated within the EOM 2.0 framework [58] . Chemical cross-linking Deglycosylated and glycosylated Mt CDH and Nc CDH were diluted to a final concentration of 0.5–1 mg ml –1 with 50 mM HEPES buffer (pH 7.5). The cross-linking was performed by adding glutaraldehyde at a final concentration of 0.5% (v/v) to the diluted protein solutions. The effect of cross-linking was tested in the absence and in the presence of 1 mM EDTA. Samples were taken before adding the cross-linker as well as at t =5, 15, 30 and 60 min after adding the cross-linker. One molar Tris buffer pH 7.5 was immediately added to the samples to neutralize the cross-linker and stop the reaction, after which the samples were mixed with sample buffer and reducing agents (50 mM dithiothreitol), heated for 5 min at 75 °C, and loaded on 3–8% NuPAGE Tris Acetate gels (Life technologies). Automated molecular docking of Nc CDH-CYT and Nc LPMO 9F We performed automated molecular docking of Nc LPMO 9F and Nc CDH with the program HADDOCK 2.0 ( http://haddock.science.uu.nl/services/HADDOCK/haddock.php [59] , [60] , [61] ). The program requires suggestions for interacting regions, and two hypotheses were tested. One protocol evaluated an interaction between the previously proposed surface patch on LPMO [23] and the haem in CYT, and another protocol tested an interaction between the copper-binding surface of LPMO and haem. Only the structures of the Nc CYT domain and Nc LPMO 9F were used. Illustrations Figures were produced using the program PyMOL (DeLano, www.pymol.org ). Accession codes. Atomic coordinates and structure factor amplitudes have been deposited with the Protein Data Bank ( www.rcsb.org ) under accession codes 4QI3 ( Mt CYT), 4QI4 ( Mt DH), 4QI5 ( Mt DH-CBLM), 4QI6 ( Mt CDH), 4QI7 ( Nc CDH) and 4QI8 ( Nc LPMO 9F ). How to cite this article: Tan, T.-C. et al . Structural basis for cellobiose dehydrogenase action during oxidative cellulose degradation. Nat. Commun. 6:7542 doi: 10.1038/ncomms8542 (2015).